Structural basis for Smoothened receptor modulation and chemoresistance to anticancer drugs The Smoothened receptor (SMO) mediates signal transduction in the hedgehog pathway, which is implicated in normal development and carcinogenesis. SMO antagonists can suppress the growth of some tumours; however, mutations at SMO have been found to abolish their antitumour effects, a phenomenon known as chemoresistance. Here we report three crystal structures of human SMO bound to the antagonists SANT1 and Anta XV, and the agonist, SAG1.5, at 2.6–2.8 Å resolution. The long and narrow cavity in the transmembrane domain of SMO harbours multiple ligand binding sites, where SANT1 binds at a deeper site as compared with other ligands. Distinct interactions at D473 6.54f elucidated the structural basis for the differential effects of chemoresistance mutations on SMO antagonists. The agonist SAG1.5 induces a conformational rearrangement of the binding pocket residues, which could contribute to SMO activation. Collectively, these studies reveal the structural basis for the modulation of SMO by small molecules. The hedgehog (Hh) signal transduction network has essential roles in the maintenance of normal embryonic development and postnatal tissue integrity in many eukaryotes ranging from Drosophila to humans [1] , [2] . Aberrant activation of the Hh signalling pathway apparently both promotes carcinogenesis—particularly in basal cell carcinomas and medulloblastomas—and supports the tumour microenvironment in many other cancers [3] . The Smoothened receptor (SMO) belongs to the Frizzled Family (or class F) receptors, which is part of the G-protein-coupled receptor (GPCR) superfamily. SMO is normally negatively regulated by a catalytic amount of the 12-transmembrane domain protein Patched [4] . In the vertebrate canonical Hh signalling pathway, the binding of the Hh signalling proteins to Patched can induce the translocation of SMO to primary cilium, thereby inducing the processing of GLI transcription factors into their active forms, which subsequently undergo nuclear translocation and activate GLI-targeted genes [2] . It has been proposed that Patched acts as a transporter and controls SMO activity by controlling the availability of small molecule lipid modulators of SMO [4] . Although the identity of the endogenous small molecule modulator of SMO is unknown, a number of exogenous small molecules that modulate SMO activity have been discovered [5] . Notably, the naturally occurring teratogen cyclopamine, which was the first selective SMO ligand, inhibits Hh signalling presumably via SMO antagonism by targeting to its 7-transmembrane (7TM) domain [6] . Given the importance of inhibiting Hh signalling pathways in various cancers, small molecules that target SMO are under intensive development, and several lead compounds are currently in clinical trials, including Vismodegib (GDC-0449, Supplementary Fig. 1 ), which was approved by the US Food and Drug Administration in 2012 for treating basal cell carcinoma [7] , [8] . Despite the tremendous progress in explicating SMO pharmacology and the recent success in obtaining the first human SMO structure [9] , a molecular understanding of the structural basis for small molecule recognition of SMO remains elusive. This is not only important for understanding the structure–activity relationships of chemically distinct SMO ligands but also for providing a mechanistic understanding of chemoresistant mutations. For example, the D473 6.54f H (superscripts in X.YY format indicate residue numbering using the new class F Ballesteros–Weinstein nomenclature [10] based on residue conservation with class F receptors, as specified in Supplementary Fig. 2 ) mutation in human SMO makes antagonists such as GDC-0449 unable to inhibit the receptor [11] , while several other compounds are insensitive to this drug resistance mutation [12] , [13] , [14] . Delineating the structural basis for the differential effects of mutations on diverse ligands would provide a rational platform for the development of drugs to counteract emerging drug resistance effects. In addition, the modulation of SMO by small molecules reveals complicated effects on ligand efficacy. For example, SAG (3-chloro- N -[4-(methylamino)cyclohexyl]- N -[3-(pyridin-4-yl)benzyl]benzo[b]thiophene-2-carboxamide) [15] , [16] and derivatives including SAG1.5 (3-chloro-4,7-difluoro- N -[ trans -4-(methylamino)cyclohexyl]- N -[[3-(4-pyridinyl)phenyl]methyl]-1-benzothiophene-2-carboxamide) [16] ( Supplementary Fig. 1 ) act as potent agonists, inducing cilia translocation of SMO and GLI transcription factor activation. Cyclopamine and SANT1 ( N -[(1E)-(3,5-dimethyl-1-phenyl-1H-pyrazol-4-yl)methylidene]-4-(phenylmethyl)-1-piperazinamine) [15] ( Supplementary Fig. 1 ), for instance, both inhibit GLI transcription factor activation, while SANT1 inhibits and cyclopamine induces cilia translocation of SMO [17] . In addition, molecules such as cyclopamine and GDC-0449, which were initially discovered as potent antagonists for the canonical Hh signalling pathway, act as agonists to induce the glucose uptake response and drive Warburg-like metabolism in fat and muscle cells via a transcription factor-independent pathway [18] , perhaps accounting for the unwanted side effects of weight loss and muscle cramping observed in humans. Clearly, determining the binding modes of different ligands to SMO represents an essential first step for correlating a ligand’s chemotype with its pattern of functional modulation, thereby illuminating the pharmacology and biology of SMO. In this study, we report three crystal structures of the human SMO 7TM domain bound to SMO small molecule antagonists SANT1, Anta XV (2-(6-(4-(4-benzylphthalazin-1-yl)piperazin-1-yl)pyridin-3-yl)propan-2-ol) [19] and agonist SAG1.5 ( Supplementary Fig. 1 ). Structure-guided mutagenesis and competition binding analysis probed the specific effects of key amino-acid residues in these structures. A further examination of these structures alongside the structures of the human SMO in complex with LY2940680 (ref. 9 ) and cyclopamine [20] provides a comprehensive framework for understanding the structural basis of molecular recognition and modulation at SMO by small molecules. Crystallization and structures of SMO–ligand complexes To investigate the structural basis of activation and inhibition of SMO, we solved the structure of SMO in complex with ligands of different functional properties including the antagonists SANT1 and Anta XV, and the potent agonist SAG1.5. Using the previously reported SMO construct [9] with the N-terminal cysteine-rich domain (CRD, residues 1–189) replaced by a thermostabilized apocytochrome b 562 RIL (BRIL), and a truncated C terminus at Q555 (BRIL-ΔCRD-SMO-ΔC), we obtained crystals of SMO bound to SANT1, Anta XV and SAG1.5. 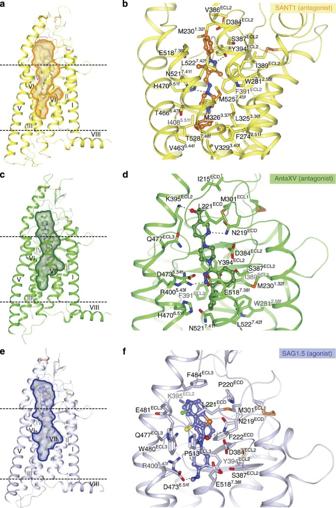Figure 1: Overall structures of SMO receptor bound to different ligands and the ligand binding pockets. (a,c,e) Overall structures of SMO receptor in complex with SANT1, Anta XV and SAG1.5, respectively. The lipid bilayer is shown in dashed lines. The ligand binding cavity is shown in surface presentation. SMO_SANT1 structure (yellow), SMO_Anta XV structure (green), and SMO_SAG1.5 structure (light blue) are shown in ribbon presentation. (b,d,f) The structures of the ligand binding pockets for SANT1 (orange carbon), Anta XV (green carbon) and SAG1.5 (light blue carbon) are shown. Polar interactions between the receptor and the ligands are shown as dashed lines and interacting residues are labelled. The structure of the SMO_SANT1 complex was solved at 2.8 Å resolution in a C222 1 space group ( Table 1 ). However, initial crystals of SMO with Anta XV and SAG1.5 diffracted to only 3.5 and 8 Å, respectively. In order to improve the resolution of the Anta XV and SAG1.5 bound SMO complexes, we applied another fusion strategy by replacing intracellular loop 3 (ICL3; from P434 to K440) with BRIL (ΔCRD-SMO-BRIL(ICL3)-ΔC). Using this construct, the structure of the SMO_Anta XV complex was solved in a P2 1 2 1 2 1 space group at 2.6 Å resolution; the structure of the SMO_SAG1.5 complex was solved in a C2 space group with resolution cutoff at 2.9, 2.5 and 3.3 Å along a*, b* and c* axes, respectively, owing to the anisotropic nature of the diffraction ( Table 1 ). In addition, we have solved the SMO_cyclopamine complex structure (PDB id: 4O9R) using a newly developed technique of serial femtosecond crystallography with lipidic cubic phase (LCP) grown crystals (LCP-SFX) at an X-ray free electron laser source. Albeit at a lower resolution, this structure unambiguously located the binding site of cyclopamine [20] . The crystal packing analysis ( Supplementary Fig. 3 ) reveals that the SMO_SANT1, SMO_Anta XV and SMO_cyclopamine complexes were crystallized as monomers, whereas the SMO_SAG1.5 complex was crystallized as a dimer, similar to the previously reported SMO_LY2940680 complex [9] (PDB id: 4JKV), with a dimer interface involving helices IV and V. Table 1 Data collection and refinement statistics. Full size table Along with the SMO_LY2940680 and SMO_cyclopamine complex structures, the newly solved structures show that the long and narrow cavity formed by the extracellular domain (ECD) linker domain, extracellular loops (ECLs) and the 7TM bundle provides multiple binding sites for small molecule ligands ( Fig. 1 and Supplementary Fig. 4 ). Similar to LY2940680 and cyclopamine, the binding sites of Anta XV and SAG1.5 are formed mostly by residues from the ECD linker domain and ECLs ( Fig. 1d,f ). In addition, Anta XV, SAG1.5 and LY2940680 form hydrogen bonds with the N219 ECD side chain, which provides an important anchor for ligands that bind close to the entrance of the ligand binding cavity. In contrast, SANT1 binds at a unique site in the cavity, which extends much deeper toward the center of the 7TM bundle and is formed mainly by residues from all the transmembrane α-helices, with the exception of helix IV ( Fig. 1b ). Figure 1: Overall structures of SMO receptor bound to different ligands and the ligand binding pockets. ( a , c , e ) Overall structures of SMO receptor in complex with SANT1, Anta XV and SAG1.5, respectively. The lipid bilayer is shown in dashed lines. The ligand binding cavity is shown in surface presentation. SMO_SANT1 structure (yellow), SMO_Anta XV structure (green), and SMO_SAG1.5 structure (light blue) are shown in ribbon presentation. ( b , d , f ) The structures of the ligand binding pockets for SANT1 (orange carbon), Anta XV (green carbon) and SAG1.5 (light blue carbon) are shown. Polar interactions between the receptor and the ligands are shown as dashed lines and interacting residues are labelled. Full size image The deep binding site of SANT1 The binding site of SANT1 is unusually deep in the 7TM helical bundle, with the ligand extending at least 9 Å deeper into the cavity compared with LY2940680 ( Fig. 2a ). The only ECL that interacts with SANT1 is ECL2, which is positioned inside the helical bundle and forms nonpolar contacts and a hydrogen bond from Y394 ECL2 to the phenyl ring and the pyrazole ring of SANT1, respectively, ( Fig. 1b ). In the helical bundle, this binding pocket is very narrow, providing a snug fit for the long and linear structure of SANT1. The side chain of H470 6.51f forms a hydrogen bond to a nitrogen in the piperazine ring ( Fig. 1b ). Superposition of the SMO_SANT1 and the SMO_SAG1.5 structures ( Fig. 2a ) reveals only a minimal overlay between SANT1 and SAG1.5, thereby providing a structural explanation for previous observations that SANT1 allosterically modulates the binding of SAG [21] , which is a close derivative of SAG1.5 ( Supplementary Fig. 1 ). In the SMO_SANT1 complex, the compound induces a slight expansion in the deep part of the cavity, as compared with the other ligands that do not reach this sub-pocket ( Fig. 2b,c ). This change in the pocket is manifested mainly in a conformational rearrangement of the side chains, while minimally affecting the protein backbone. The side chain of L325 3.36f protrudes into the central cavity when this deep pocket is not occupied, but rotates out from the cavity making space for the binding of SANT1 ( Fig. 2d ). In addition, the side chain of M525 7.45f moves towards SANT1 to make contact with the piperazine moiety of the ligand. To further investigate the binding pocket for SANT1, we introduced bulky side-chain mutations, L325 3.36f F, V329 3.40f F, I408 5.51f F and T466 6.47f Q, in the bottom part of the pocket ( Fig. 2d ), aiming to block this binding site without disturbing the overall receptor conformation. While the binding of the radioligand 3 H-cyclopamine remains unchanged in agreement with the SMO_cyclopamine structure, competition radioligand binding experiments reveals that three of these bulky mutations, V329 3.40f F, I408 5.51f F and T466 6.47f Q, substantially reduce the binding of SANT1 ( Fig. 2e and Supplementary Table 1 ). Interestingly, the L325 3.36f F mutation has no effect on SANT1 binding, consistent with the modelling of the L325 3.36f F mutation that shows that the SMO_SANT1 complex can easily accommodate a phenyl side chain in the rotamer state observed for L325 3.36f in the SANT1 bound structure ( Fig. 2d ). Binding of the other tested ligands was not substantially affected by any of these bulky side-chain mutations ( Fig. 2e ), corroborating the unique nature of the deep binding site for SANT1 among the other SMO ligands studied. 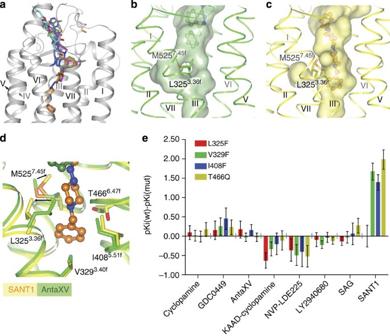Figure 2: The deep binding pocket of SANT1. (a) Localization of different ligands in the binding pocket: SANT1 (orange), Anta XV (green), SAG1.5 (light blue), LY2940680 (magenta) and cyclopamine (cyan). (b,c) The shapes of the deep binding pockets in the structures of SMO_Anta XV (green) and SMO_SANT1 (yellow), respectively. (d) Superposition of the deep binding pockets in the structures of SMO_Anta XV and SMO_SANT1. The side-chain movements induced by SANT1 binding are shown by arrows. (e) ΔpKi values (pKi wild-type (wt)–pKi mutants (mut)) of the designed mutants for different SMO ligands in3H-cyclopamine competition experiments. Shown in the graph are mean±s.e.m. of 3–4 independent experiments, see alsoSupplementary Table 1. Figure 2: The deep binding pocket of SANT1. ( a ) Localization of different ligands in the binding pocket: SANT1 (orange), Anta XV (green), SAG1.5 (light blue), LY2940680 (magenta) and cyclopamine (cyan). ( b , c ) The shapes of the deep binding pockets in the structures of SMO_Anta XV (green) and SMO_SANT1 (yellow), respectively. ( d ) Superposition of the deep binding pockets in the structures of SMO_Anta XV and SMO_SANT1. The side-chain movements induced by SANT1 binding are shown by arrows. ( e ) ΔpKi values (pKi wild-type (wt)–pKi mutants (mut)) of the designed mutants for different SMO ligands in 3 H-cyclopamine competition experiments. Shown in the graph are mean±s.e.m. of 3–4 independent experiments, see also Supplementary Table 1 . Full size image The binding mode of cyclopamine and KAAD–cyclopamine The naturally occurring steroidal jerveratrum alkaloid cyclopamine was the first small molecule found to bind to and inhibit Hh signalling via SMO. Cyclopamine binds close to the extracellular entrance, and the secondary amine of its 3-methyl-piperidine group points outside of the pocket, whereas the 3,β-hydroxyl is buried deep in the pocket ( Supplementary Fig. 5a ) [20] . This binding pose is consistent with previous structure–activity relationship studies of cyclopamine derivatives, which showed that adducts to the 3,β-hydroxyl markedly reduced activity, while the secondary amine permits addition of bulky groups via long aliphatic linkers [22] . One such molecule is KAAD–cyclopamine (3-keto- N -(aminoethyl-aminocaproyl-dihydrocinnamoyl)cyclopamine) ( Supplementary Fig. 1 ), which is derived by attaching a long-chain substitution to the secondary amine of cyclopamine. Our data show that the binding of KAAD–cyclopamine to SMO is not impacted by mutations blocking the deep binding pocket ( Fig. 2e ), consistent with a predicted binding mode where the long-chain substitution extends out of the 7TM cavity through the extracellular ligand entrance ( Supplementary Fig. 5b ). The long aliphatic linker protruding out of the pocket has also been shown to enable attachments as large as a fluorescent BODIPY (boron-dipyrromethene) moiety to cyclopamine [6] . Differential binding modes of Anta XV and LY2940680 Although Anta XV and LY2940680 share a phthalazine ring core and a similar overall shape, different substitutions on the phthalazine ring result in distinct binding modes of these ligands. In the previously solved SMO_LY2940680 structure [9] , the 4-fluoro-2-trifluoromethylphenyl moiety of LY2940680 forms extensive interactions with residues from ECL3, including Q477, W480, E481 and F484, which stacks to the phenyl ring of LY2940680 through a π – π interaction ( Fig. 3a ). In contrast, Anta XV does not have contacts with ECL3, and the side-chain residue conformations of ECL3 in the SMO_Anta XV structure are more similar to those in the structure of SMO_SANT1, which also lacks ECL3 contacts ( Supplementary Fig. 6 ). The differential interaction of LY2940680 with ECL3 apparently results in an overall shift of the α-helical portion of ECL3 ( Fig. 3b,c ). 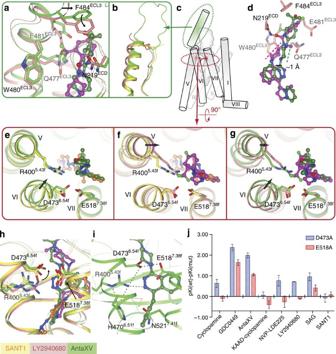Figure 3: D4736.54fhas different roles in the recognition of Anta XV and LY2940680. (a–i) The receptor structures in SMO_Anta XV, SMO_SANT1 and SMO_LY2940680 (PDB i.d.: 4JKV, molecule A) complexes are shown in green, yellow and salmon, respectively. Ligand structures of Anta XV, SANT1 and LY2940680 are shown in green, orange and magenta carbons, respectively. (a) Superposition of SMO_LY2940680 and SMO_Anta XV structures near ECL3. The conformational change of F484ECL3induced by LY2940680 binding is shown by an arrow. See alsoSupplementary Fig. 5for comparison with SMO_SANT1 structure. (b) Superposition of the SMO_SANT1, SMO_Anta XV and SMO_LY2940680 structures reveals a different conformation of ECL3 in LY2940680 bound structure (shown by arrow). (c) Localization of ECL3 (green) and polar residue cluster (R4005.43f, D4736.54fand E5187.38f, red) in SMO. (d) Superposition of the binding poses of LY2940680 and Anta XV reveals distinct orientations (dashed lines parallel to the equatorial bonds of the six-membered chair conformation rings) of the six-membered rings connected to the phthalazine ring. The shift of the phthalazine of LY2940680 compared with that of Anta XV is shown by arrow. (e) Superposition of SMO_Anta XV and SMO_SANT1 structures. (f) Superposition of SMO_LY2940680 and SMO_SANT1 structures. (g) Superposition of SMO_LY2940680 and SMO_Anta XV structures. Ligand-induced shifts of helices are shown by arrows. (h) Superposition of the ligand binding pocket residues of SMO_SANT1, SMO_Anta XV and SMO_LY2940680 structures. Ligand interaction-induced conformation change at D4736.54fis indicated by arrow. (i) Polar residue cluster in the ligand binding pocket of the SMO_Anta XV structure. Polar interactions are shown as dashed lines. (j) ΔpKi values (pKi wild-type(wt)–pKi mutants (mut)) of the D4736.54fA and E5187.38fA mutants for different SMO receptor ligands in3H-cyclopamine competition experiments. Shown in the graph are mean±s.e.m. of 3–4 independent experiments, see alsoSupplementary Table 2. Figure 3: D473 6.54f has different roles in the recognition of Anta XV and LY2940680. ( a – i ) The receptor structures in SMO_Anta XV, SMO_SANT1 and SMO_LY2940680 (PDB i.d. : 4JKV, molecule A) complexes are shown in green, yellow and salmon, respectively. Ligand structures of Anta XV, SANT1 and LY2940680 are shown in green, orange and magenta carbons, respectively. ( a ) Superposition of SMO_LY2940680 and SMO_Anta XV structures near ECL3. The conformational change of F484 ECL3 induced by LY2940680 binding is shown by an arrow. See also Supplementary Fig. 5 for comparison with SMO_SANT1 structure. ( b ) Superposition of the SMO_SANT1, SMO_Anta XV and SMO_LY2940680 structures reveals a different conformation of ECL3 in LY2940680 bound structure (shown by arrow). ( c ) Localization of ECL3 (green) and polar residue cluster (R400 5.43f , D473 6.54f and E518 7.38f , red) in SMO. ( d ) Superposition of the binding poses of LY2940680 and Anta XV reveals distinct orientations (dashed lines parallel to the equatorial bonds of the six-membered chair conformation rings) of the six-membered rings connected to the phthalazine ring. The shift of the phthalazine of LY2940680 compared with that of Anta XV is shown by arrow. ( e ) Superposition of SMO_Anta XV and SMO_SANT1 structures. ( f ) Superposition of SMO_LY2940680 and SMO_SANT1 structures. ( g ) Superposition of SMO_LY2940680 and SMO_Anta XV structures. Ligand-induced shifts of helices are shown by arrows. ( h ) Superposition of the ligand binding pocket residues of SMO_SANT1, SMO_Anta XV and SMO_LY2940680 structures. Ligand interaction-induced conformation change at D473 6.54f is indicated by arrow. ( i ) Polar residue cluster in the ligand binding pocket of the SMO_Anta XV structure. Polar interactions are shown as dashed lines. ( j ) ΔpKi values (pKi wild-type(wt)–pKi mutants (mut)) of the D473 6.54f A and E518 7.38f A mutants for different SMO receptor ligands in 3 H-cyclopamine competition experiments. Shown in the graph are mean±s.e.m. of 3–4 independent experiments, see also Supplementary Table 2 . Full size image Together with the extensive interactions between the 4-fluoro-2-trifluoromethylphenyl group of LY2940680 and ECL3, the hydrogen bond between N219 and the carbonyl group of LY2940680 potentially defines the orientation of piperidine ring substituent on the phthalazine core, which is distinct from the orientation of the piperazine ring of Anta XV ( Fig. 3d ). In this orientation, the phthalazine core of LY2940680 adopts an axial position in the chair conformation of the six-membered piperidine ring, which was estimated to be slightly (ΔE~0.72 kcal mol −1 ; ref. 23 ) suboptimal compared with the equatorial position. In contrast, on the piperazine ring of Anta XV, the phthalazine core sits in the equatorial position; this difference in ring conformation is accompanied by a 1-Å shift of the phthalazine ring between the two ligands ( Fig. 3d ). The shift is also associated with a shift at the guanidinium group of R400 5.43f that forms a hydrogen bond to the phthalazine core of Anta XV and LY2940680, as well as the extracellular end of helix V where R400 5.43f is located ( Fig. 3e–g ). This difference in the positions of the phthalazine core in Anta XV and LY2940680 may explain their distinctive interactions with D473 6.54f , a key residue in a polar interaction cluster within the ligand binding cavity ( Fig. 3c,i ). First, the side chain of D473 6.54f makes a direct interaction with Anta XV (3.3 Å), whereas its interaction with LY2940680 is much weaker as revealed by a longer distance (4.0 Å in molecule A and 4.3 Å in molecule B). Second, the interaction between D473 6.54f and Anta XV is accompanied by an inward shift of the extracellular tip of helix VI, as compared with SMO_SANT1 and SMO_LY2940680 structures where their respective ligands do not interact with D473 6.54f ( Fig. 3e–g ). The difference in this interaction is also reflected in different rotamer states of the carboxylate group of D473 6.54f ( Fig. 3h ). All these structural data point to a more important role for D473 6.54f in Anta XV recognition compared with LY2940680. Mutation of D473 6.54f into histidine has been identified as a cause of chemoresistance for GDC-0449, while LY2940680 has been reported to be unaffected by this mutation [24] . To investigate the role of D473 6.54f in the binding of different ligands, we performed 3 H-cyclopamine competition binding assays on a D473 6.54f A mutant, as well as an E518 7.38 A mutant that could impact the conformation of D473 6.54f . The natural drug-resistance mutation D473 6.54f H and other mutations that could impact the conformation of D473 6.54f , such as R400 5.43f A, H470 6.51f A and N521 7.41f A ( Fig. 3h ), unfortunately could not be assessed in the radioligand competition assay, as they abolished the binding of radioligand 3 H-cyclopamine. Among the mutations that retained binding of the radioligand, the D473 6.54f A and E518 7.38f A mutations impaired the binding of GDC-0449 and Anta XV, with D473 6.54f A responsible for a >100-fold affinity drop for both ligands. In contrast, the effect of D473 6.54f A mutation on LY2940680 was modest (<7-fold), consistent with the lack of such a direct interaction in the SMO_LY2940680 structure ( Fig. 3j and Supplementary Table 2 ). Moreover, these mutations have no effect on the binding of SANT1, which is consistent with the fact that in the SMO_SANT1 structure D473 6.54f has little role in ligand binding. These results thus provide a direct structural explanation for the differential effect of ligand binding pocket mutations on ligands with distinct binding poses. Remodelling of the SMO binding pocket by agonist SAG1.5 When bound to SMO, the two aromatic rings of SAG1.5 pack against each other, forming a bulky system that fits tightly into the pocket surrounded by the ECD linker domain and ECLs close to the extracellular entrance ( Fig. 1f ). This clamping of the bulky aromatic groups of SAG1.5 by the ECL structures points the cyclohexane deeper into the 7TM bundle, aligning the positively charged methyl amino group in the vicinity of polar residue cluster, R400 5.43f , D473 6.54f and E518 7.38f ( Figs 1f and 4 ), which are the only residues from the seven helixes that interact with the agonist. In the antagonist bound structures, the D473 6.54f and E518 7.38f side chains point towards each other and interact directly, or in the case of the SMO_LY2940680 structure, through water-mediated interactions. In the agonist bound structure, the positively charged amino group of SAG1.5 forms an ionic interaction with D473 6.54f , whereas the carboxyl group of E518 7.38f moves away and no longer interacts with D473 6.54f ( Fig. 4a ). In the antagonist bound structures, R400 5.43f is anchored by polar interactions with D473 6.54f , H470 6.51f and/or the ligands. In the agonist bound structure, the guanidine group of R400 5.43f moves up to form a hydrogen bond with the side chain of Q477 ECL3 ( Fig. 4b ). This remodelling at the residues R400 5.43f , D473 6.54f and E518 7.38f ( Fig. 4c ) is the most pronounced change in the ligand binding pocket, differentiating the SMO_SAG1.5 structure from the antagonist bound structures. In addition, subtle modifications at the amino group of the SAG scaffold have been shown to change the functional property of the ligand, that is, from agonist to antagonist [25] , indicating that this amino group has a critical role in the SMO modulation by SAG1.5. Although previous studies showed that oxysterol binding at the N terminus of SMO can induce activation [26] , [27] , [28] , the SAG1.5 bound SMO structure reveals an alternative site at the 7TM domain that is responsible for the small molecule-induced activation of the receptor ( Fig. 5 ). 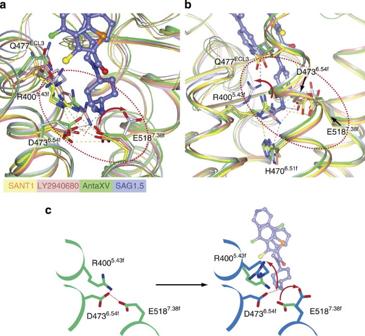Figure 4: Agonist SAG1.5-induced conformational changes in the ligand binding pocket. (a) Superposition of the ligand binding pocket residues of different structures of SMO. The receptor structure and side-chain carbons are shown for SMO_Anta XV (green), SMO_SANT1 (yellow), SMO_LY2940680 (salmon; PDB i.d.: 4JKV, molecule A), and SMO_SAG1.5 (light blue) structures. The ligand SAG1.5 is shown as light blue carbons. The hydrogen bond interactions between side chains are show as dashed lines in the corresponding colour of each structure. (b) A different view of the superposition of the ligand binding pocket residues. H4706.51fthat interacts with R4005.43fin antagonist bound structures is shown. Red arrows (ina,b) are shown to indicate the conformational changes of E5187.38fand R4005.43finduced by SAG1.5 binding. (c) Schematic presentation of agonist-induced conformation change: green is antagonist bound state, whereas blue is agonist bound state. Figure 4: Agonist SAG1.5-induced conformational changes in the ligand binding pocket. ( a ) Superposition of the ligand binding pocket residues of different structures of SMO. The receptor structure and side-chain carbons are shown for SMO_Anta XV (green), SMO_SANT1 (yellow), SMO_LY2940680 (salmon; PDB i.d. : 4JKV, molecule A), and SMO_SAG1.5 (light blue) structures. The ligand SAG1.5 is shown as light blue carbons. The hydrogen bond interactions between side chains are show as dashed lines in the corresponding colour of each structure. ( b ) A different view of the superposition of the ligand binding pocket residues. H470 6.51f that interacts with R400 5.43f in antagonist bound structures is shown. Red arrows (in a , b ) are shown to indicate the conformational changes of E518 7.38f and R400 5.43f induced by SAG1.5 binding. ( c ) Schematic presentation of agonist-induced conformation change: green is antagonist bound state, whereas blue is agonist bound state. 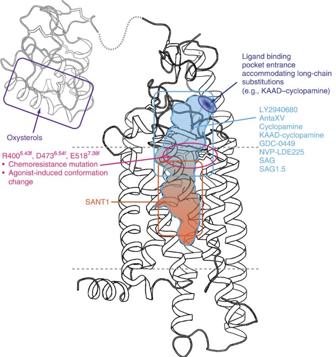Figure 5: Map of the structural basis for the modulation of SMO by small molecules. The N-terminal CRD is shown using the CRD of zebrafish SMO (PDB i.d.: 4C79). The boundaries of the membrane bilayer are shown as dashed lines. Full size image Figure 5: Map of the structural basis for the modulation of SMO by small molecules. The N-terminal CRD is shown using the CRD of zebrafish SMO (PDB i.d. : 4C79). The boundaries of the membrane bilayer are shown as dashed lines. Full size image On the intracellular side, the most pronounced difference between agonist and antagonist bound structures is observed at Y262 ICL1 , H361 4.46f and W365 4.50f that are conserved among class F receptors [9] . In all the antagonist bound structures, we observed a hydrogen bonding network among these residues. In the agonist bound structure, the hydrogen bond between Y262 ICL1 and H361 4.46f is broken, which is associated with an inward movement of P263 ICL1 , which is also conserved among class F receptors [9] , to make contact with W535 7.55f ( Supplementary Fig. 7 ). Mutation of W535 7.55f into leucine has been shown to make the SMO receptor constitutively active leading to carcinogenesis [29] . In addition, W535 7.55f is located at the intracellular end of helix VII, immediately adjacent to helix VIII ( Supplementary Fig. 7 ), which packs against helix I, and parallel to the membrane layer, and has an important role during the activation of SMO since mutation at the residues W545 and R546 located in helix VIII impairs cilia translocation [30] . These conformational changes observed at Y262 ICL1 , H361 4.46f , W365 4.50f and P263 ICL1 could impact W535 7.55f , and are conceivably important for SMO activation. We note, however, that the change of the hydrogen bond state could result from the slightly lower pH in the crystallization condition of the agonist bound receptor. Thus, the involvement of this conformational change during SMO activation needs to be investigated in future studies. With the exception of this local conformational change, the agonist SAG1.5 bound SMO structure does not show any large-scale movements in helices VI and VII, which are the hallmark of class A GPCR activation [31] . This may be because of the stark differences in signalling mechanisms between the two GPCR classes, or the possibility that in the absence of downstream effectors SAG1.5 induces only part of the activation-related conformational changes in SMO or other factors (see Discussion section). The newly solved structures of SMO bound to SANT1, Anta XV and SAG1.5, along with the LY2940680 and cyclopamine bound structures, reveal a variety of distinctive poses for structurally diverse small molecule ligands in the long and narrow cavity defined by the 7TM helices, ECD and ECLs of SMO ( Fig. 5 ). The antagonist SANT1, for instance, binds very deep in the pocket, whereas the other ligands studied remain closer to the extracellular entrance, demonstrating that the entire long and narrow pocket can be targeted by small molecule ligands. Meanwhile, the extracellular entrance can provide a path for accommodating the attachment of reporter moieties or other bulky groups to the ligands through a long-chain flexible linker such as that of KAAD–cyclopamine. Even when the binding sites largely overlap, as for instance with LY2940680 and Anta XV, minor differences in recognition modes result in a discrete response to binding pocket mutations. LY2940680, for example, has been reported to bind the D473 6.54f H mutant that provides chemoresistance to the approved cancer drug GDC-0449 (ref. 24 ). This biological phenomenon accords nicely with our structural analysis that shows that LY2940680 forms weak interactions with D473 6.54f . In contrast, the binding of Anta XV requires a more substantial involvement of D473 6.54f , as revealed by the structural and mutagenesis data, despite its similar scaffold with LY2940680. The most striking difference between the binding mode of LY2940680 and Anta XV is a strong interaction between LY2940680 and ECL3. We hypothesize that this interaction restrains the orientation of LY2940680, which leads to a shift of the phthalazine core of LY2940680 away from D473 6.54f compared with Anta XV, weakening the role of D473 6.54f in ligand binding. This reduced involvement of D473 6.54f in binding might also underlie the effect of chemical modifications on existing compounds that could overcome the drug-resistant mutation D473 6.54f H as shown in studies with derivatives of GDC-0449 (ref. 12 ) and Anta XV (ref. 14 ). The long and continuous cavity straddling the ECL region and 7TM domain of SMO provides a variety of binding sub-sites suitable for ligand interaction. Taken together, this structural information should facilitate the development of compounds, which bypass this chemoresistant mutation or have a larger contacting surface so that disruption of a local structure, as chemoresistance mutations do, could not abolish the ligand binding. We observed remodelling of the polar interaction network between R400 5.43f , D473 6.54f and E518 7.38f in the binding pocket induced by SAG1.5; such remodelling could conceivably serve as an activation trigger. However, because of the lack of knowledge regarding the immediate biochemical events downstream of SMO 7TM domain activation, a mechanistic connection between the ligand-triggered activation at the extracellular side and the intracellular coupling with downstream proteins remains to be established. SMO has shown in some studies an ability to activate G-proteins [32] that presumably requires an opening of the intracellular crevice for G-protein binding [33] as has been established in class A GPCRs. Some conformationally selective ligands are capable of converting class A GPCRs into a partially activated state where the change in the ligand binding pocket propagates into the intracellular side of the receptors [34] , [35] , [36] , [37] , [38] . In other cases, for example, in β-adrenergic receptors, agonist binding alone is insufficient for stabilization of an active state, and therefore in the structures of these receptors obtained in the absence of G-proteins or their mimetics the intracellular side maintains the inactive conformation [39] , [40] . In the SAG1.5 bound SMO structure, we did not observe the remodelling of the intracellular side that has been demonstrated in the active state class A GPCR structures. This could be because of the following reasons: (i) although SAG1.5 is a potent agonist for the canonical Hh signalling pathway, it is not an effective agonist for G-protein activation; (ii) the insertion of BRIL at ICL3 prevented intracellular helical movement; and (iii) conformational changes at the intracellular part of the receptor require binding of G-proteins as observed for β-adrenergic receptors. Owing to the divergence of the canonical Hh signalling pathway from the traditional G-protein pathway, it is possible that the activated SMO couples to as yet unidentified intracellular effector(s) that could eventually elicit conformational changes responsible for an active state. Alternatively, activation by agonist might induce only small conformational changes in the 7TM domain, which modify oligomerization states or lead to differential association with membrane compartments and intracellular trafficking machineries. This long and narrow cavity responsible for the binding of small molecule ligands investigated in this study is not the only modulation site for SMO. Lipid molecules have been shown to be able to modulate SMO, for example, cholesterol depletion severely impairs SMO activation [26] . It has been suggested that the endogenous modulation mechanism of SMO by Patched might also be mediated through a lipidic molecule [4] . Oxysterols, for instance, have been shown to activate SMO and had been suspected to be native ligands for SMO. However, recent studies showed that oxysterols bind to the N-terminal CRD ( Fig. 5 ), the structure of which has been solved by crystallography [27] and nuclear magnetic resonance [41] methods, and that the CRD is important, but not essential, for the Hh-induced activation of SMO as well as for cholesterol dependence of Hh signalling [26] , [27] , [28] . Thus, there could be additional sites in the 7TM domain that serve as the binding sites of native modulators or lipidic molecules. A previous study showed that mutations within the ligand binding site that disrupt binding of synthetic ligands, such as cyclopamine, fail to impair the normal basal and Hh-induced activity, as well as the cholesterol dependence of Hh signalling [26] , indicating that an alternative site might be used to modulate SMO activity by Patched or lipidic molecules. W 4.50 has been shown to be a conserved lipid binding site at class A GPCRs [42] , [43] , [44] that locates at the interface between the 7TM domain and membrane environment, and is thus accessible to lipidic molecules. In the agonist bound structure, we observed conformational changes in a hydrogen bond network involving W365 4.50f ( Supplementary Fig. 7 ), which occur in the vicinity of W535 7.55f , a critical residue for SMO activation. Further studies will be needed to fully investigate the role of this region in the modulation of SMO by lipidic molecules. In summary, we provide new insights into the conformational plasticity of SMO–ligand interactions by crystallographic and biochemical characterization of several SMO complexes with diverse ligand chemotypes. Importantly, these ligands target distinct sites in the elongated cavity, have different interactions with known resistance mutants and include both antagonists and agonists of Hh signalling. The details of these interactions and ligand-dependent conformational changes, correlated with specific functional features of the ligands, will help to design new clinical candidates targeting SMO with attenuated side effects and chemoresistance. Generation of BRIL–SMO fusion constructs. The BRIL-ΔCRD-SMO-ΔC construct has been reported previously [9] . For ΔCRD-SMO-BRIL(ICL3)-ΔC, BRIL was fused to the human SMO receptor 7TM domain (S190-Q555) by replacing ICL3 residues P434 to K440 using overlapping PCR. The resulting receptor chimera sequence was subcloned into a modified pFastBac1 vector (Invitrogen), designated as pFastBac1-833100, which contained an expression cassette with a haemagglutinin signal sequence followed by a Flag tag, a 10 × His tag, and a TEV protease recognition site at the N terminus before the receptor sequence. Subcloning into the pFastBac1-833100 was achieved using PCR with primer pairs encoding restriction sites Kpn I at the 5′ and Hin dIII at the 3′ termini, with subsequent ligation into the corresponding restriction sites in the vector. Expression and purification of SMO constructs The SMO constructs were expressed in Spodoptera frugiperda ( Sf 9) insect cells using the Bac-to-Bac Baculovirus Expression System (Invitrogen). Sf 9 cells at cell density of 2-3 × 10 6 cells per ml were infected with baculovirus at 27 °C. Cells were harvested by centrifugation at 48 h post infection and stored at −80 °C until use. Insect cell membranes were lysed by thawing frozen cell pellets in a hypotonic buffer containing 10 mM HEPES, pH 7.5, 10 mM MgCl 2 , 20 mM KCl and EDTA-free complete protease inhibitor cocktail tablets (Roche). Extensive washing of the raw membranes was performed by repeated centrifugation two-three times in a high osmotic buffer comprising of 1.0 M NaCl in the hypotonic buffer described above. The washed membranes were resuspended into buffer containing 30 μM ligand, 2 mg ml −1 iodoacetamide (Sigma) and EDTA-free complete protease inhibitor cocktail tablets, and incubated at 4 °C for 1 h before solubilization. The membranes were then solubilized in buffer containing 50 mM HEPES, pH 7.5, 200 mM NaCl, 1% (w/v) n -dodecyl-β-D-maltopyranoside (DDM; Anatrace), 0.2% (w/v) cholesteryl hemisuccinate (CHS; Sigma), 15 μM ligand, for 3–4 h at 4 °C. The supernatant containing solubilized SMO protein was isolated from the cell debris by high-speed centrifugation, and subsequently incubated with TALON IMAC resin (Clontech) overnight at 4 °C in the presence of 20 mM imidazole and 1 M NaCl. After binding, the resin was washed with 10 column volumes of Wash I Buffer comprising of 50 mM HEPES, pH 7.5, 800 mM NaCl, 10% (v/v) glycerol, 0.1% (w/v) DDM, 0.02% (w/v) CHS, 8 mM ATP, 20 mM imidazole, 10 mM MgCl 2 and 15 μM ligand, followed by 6 column volumes of Wash II Buffer comprising 50 mM HEPES, pH 7.5, 500 mM NaCl, 10% (v/v) glycerol, 0.05% (w/v) DDM, 0.01% (w/v) CHS, 50 mM imidazole and 20 μM ligand. The protein was then eluted by 3 column volumes of Elution Buffer containing 50 mM HEPES, pH 7.5, 300 mM NaCl, 10% (v/v) glycerol, 0.03% (w/v) DDM, 0.006% (w/v) CHS, 250 mM imidazole and 50 μM ligand. PD MiniTrap G-25 column (GE Healthcare) was used to remove imidazole. The protein was then treated overnight with TEV protease (His-tagged) to cleave the N-terminal His-tag and FLAG-tag. TEV protease and cleaved N-terminal fragment were removed by TALON IMAC resin incubation at 4 °C for 2 h. The tag-less protein was collected as the TALON IMAC column flow-through. The protein was then concentrated to 50–60 mg ml −1 with a 100 kDa cutoff Vivaspin concentrator. Protein monodispersity was tested by analytical size-exclusion chromatography. Typically, the analytical size-exclusion chromatography profile showed a monodisperse peak. SANT1 ligand was purchased from Tocris Biosciences (purity >99%); Anta XV (originally named Hh Signalling Antagonist XV) ligand was purchased from Calbiochem (purity 98.94%); and SAG1.5 ligand was purchased from Xcess Biosciences Inc. (purity>98%). LCP crystallization Protein samples of SMO in a complex with certain ligand were reconstituted into LCP by mixing with molten lipid (monoolein and cholesterol mixture in a ratio of 9:1 (w/w)) in a mechanical syringe mixer [45] . LCP crystallization trials were performed using an NT8-LCP crystallization robot (Formulatrix) as previously described [46] . Ninety-six-well glass sandwich plates (Marienfeld) were incubated and imaged at 20 °C using an automated incubator/imager (RockImager 1000, Formulatrix). Crystals of SMO_SANT1 complex were grown in the following conditions: 150 mM NH 4 F, 100 mM HEPES, pH 6.9, 27% polyethylene glycol (PEG) 400 and 2.5% Jeffamine; crystals of SMO_Anta XV complex were grown in the following conditions: 100–115 mM NH 4 Cl, 100 mM HEPES, pH 7.2, and 36% PEG 400; and crystals of SMO_SAG1.5 complex were grown in the following conditions: 100 mM MgSO 4 , 100 mM 2-(N-morpholino)ethanesulfonic acid (MES), pH 6.0, 30% PEG 400 and 2–3% polypropylene glycol P 400. Crystals were harvested using MiTeGen micromounts and flash-frozen in liquid nitrogen for data collection. Crystallographic data collection and processing X-ray data were collected at the 23ID-D beamline (GM/CA CAT) at the Advanced Photon Source, Argonne, IL using a 20-μm minibeam at a wavelength of 1.0330 Å and a MarMosaic 300 CCD detector. Crystals were aligned and data were collected using strategy similar to other GPCR structures [47] . Typically 20 frames at 1° oscillation and 1 s exposure with non-attenuated beam followed by a translation of the crystal to a non-exposed position or changing the crystal to minimize the effect of radiation damage. A complete data set was obtained by indexing, integrating, scaling and merging data using HKL2000 (ref. 48 ). The SMO_SAG1.5 data set was highly anisotropic. The merged data were submitted to the UCLA anisotropy server ( http://services.mbi.ucla.edu/anisoscale ) and anisotropically truncated at 2.9, 2.5 and 3.3 Å along a*, b* and c* axes, respectively. Structure determination and refinement Initial phase information was obtained by molecular replacement with the programme PHASER [49] using two independent search models of SMO 7TM domain and BRIL from SMO_LY2940680 complex structure (PDB i.d. : 4JKV). All refinements were performed with REFMAC5 (ref. 50 ) and autoBUSTER [51] followed by manual examination and rebuilding of the refined coordinates in the programme COOT [52] using both |2F O |–|F C | and |F O |–|F C | maps, as well as omit maps calculated using the Bhat’s procedure [53] , [54] . The structures have been deposited in the PDB with the accession codes: 4N4W for SMO_SANT1 complex; 4QIM for SMO_AntaXV complex; and 4QIN for SMO_SAG1.5 complex. Radioligand competition Radioligand binding assays used crude HEK 293T membrane preparations expressing wild-type or mutant human SMO in 96-well plates at a final volume of 125 μl. To obtain crude HEK 239T membrane preparations, HEK 293T cells were transfected with wild-type or mutant human SMO expression plasmids for 24 h and scraped into conical centrifuge tubes. Collected cells were centrifuged at 1,000g for 10 min and the cell pellet was hypotonically lysed by cold lysis buffer (50 mM Tris-HCl, pH 7.4). Crude membrane fractions were isolated by centrifugation at 21,000g for 20 min at 4°C. The membrane pellets were re-suspended with lysis buffer at 3X volume of pellet size, subjected to protein concentration determination, and stored in aliquots at −80°C if not used immediately. To determine equilibrium dissociation constant (K d ) for 3 H-cyclopamine, a serial of eight concentrations of 3 H-cyclopamine (0.2–36 nM in triplicate) were incubated with 20 μg of above SMO HEK 293T membranes in binding buffer (50 mM HEPES, 3 mM MgCl 2 , EDTA-free protease inhibitor cocktail, 0.5 mg ml −1 BSA, pH 7.2) for 2.5 h in the dark at 20°C. Nonspecific binding was defined by 10 μM SMO receptor antagonist LY2940680. To determine equilibrium dissociation constant (K i ) for varies ligands, a serial of 11 concentrations of test compound (0.1 nM to 10 μM in triplicate sets) were incubated with a fixed concentration of 3 H-cyclopamine (~K d of 3 H-cyclopamine) and SMO HEK293 T membranes for 2.5 h in the dark at 20°C. At the end of the incubation period, the reactions were stopped by rapid filtration onto 0.3% PEI-soaked GF/A filters and washed three times with cold PBS (pH 7.2). The filters were then microwave dried and scintillant was melted on the filters on a hot plate. The filters were wrapped in plastic wrap and counted for radioactivity. Molecular modelling and KAAD–cyclopamine docking Conformational modelling and evaluation of the mutation effects in SMO complexes with different ligands was performed using an all-atom global energy optimization algorithm in ICM-Pro 3.7 (MolSoft LLC) molecular modelling package [55] . Point mutations of interest (L325 3.36f F, V329 3.40f F, I408 5.51f F and T466 6.47f Q) in each of the co-crystal structures were introduced by modifying the residue side chain, followed by energy optimization that included the ligand and side chains within 6 Å distance of the mutated residue. Other side chains and the backbone of the protein were kept as in the crystal structure. The effect of the mutation was evaluated by comparing conformational energy of the ligand before and after mutation. Docking of KAAD–cyclopamine was performed with all atom energy-based docking procedure with side-chain flexibility in the binding pocket [56] using the SMO_cyclopamine crystal structure. An initial conformation of KAAD–cyclopamine was generated by Cartesian optimization of the ligand model in Merck Molecular Force Field. All calculations were repeated at least in three independent runs, performed on a 12-core Intel Xeon 2.67 GHz Linux workstation. How to cite this article: Wang, C. et al. Structural basis for Smoothened receptor modulation and chemoresistance to anticancer drugs. Nat. Commun. 5:4355 doi: 10.1038/ncomms5355 (2014).